Crystalline silica-induced leukotriene B4-dependent inflammation promotes lung tumour growth Chronic exposure to crystalline silica (CS) causes silicosis, an irreversible lung inflammatory disease that may eventually lead to lung cancer. In this study, we demonstrate that in K-ras LA1 mice, CS exposure markedly enhances the lung tumour burden and genetic deletion of leukotriene B4 receptor-1 (BLT1 −/− ) attenuates this increase. Pulmonary neutrophilic inflammation induced by CS is significantly reduced in BLT1 −/− K-ras LA1 mice. CS exposure induces LTB 4 production by mast cells and macrophages independent of inflammasome activation. In an air-pouch model, CS-induced neutrophil recruitment is dependent on LTB 4 production by mast cells and BLT1 expression on neutrophils. In an implantable lung tumour model, CS exposure results in rapid tumour growth and decreased survival that is attenuated in the absence of BLT1. These results suggest that the LTB 4 /BLT1 axis sets the pace of CS-induced sterile inflammation that promotes lung cancer progression. This knowledge may facilitate development of immunotherapeutic strategies to fight silicosis and lung cancer. Lung cancer is the single largest cause of cancer-related deaths worldwide. Chronic inflammation considered the seventh hallmark of cancer is promoted by a variety of intrinsic and extrinsic factors [1] , [2] , [3] . Intrinsic factors such as activating mutation of K-ras, often associated with human lung adenocarcinomas [4] induces a pro-inflammatory microenvironment [5] . Extrinsic factors such as cigarette smoke or air-borne pollutants, commonly encountered in the environment, also promote chronic lung inflammation and cancer [6] , [7] . Exposure to air-borne particulates such as crystalline silica (CS) is a major global occupational health hazard [8] encountered in a diverse array of industrial settings such as mining, pottery, glass and concrete production. Around two million US workers and several million more worldwide are occupationally exposed to CS particles. CS exposure leads to lung infiltration of neutrophils, macrophages and lymphocytes causing lung inflammation and the problem is further compounded by massive lung fibrosis leading to the disease silicosis [9] , [10] . Silicosis is irreversible and incurable due to impaired particle clearance, resulting in persistent lung inflammation and may eventually lead to lung cancer [11] , [12] . Epidemiological data suggest that smokers with silicosis are at even higher risk of lung cancer [13] , [14] . Although the association of silicosis with lung cancer has been suspected for many decades, there were no established model systems to study mechanisms that link CS-induced chronic inflammation to lung cancer promotion. Chemokines orchestrate a tightly regulated process of inflammatory cell recruitment to sites of tissue damage, which is a key step in the process of cancer-related inflammation [15] , [16] . The lipid chemoattractant leukotriene B 4 (LTB 4 ) is one of the early mediators of inflammation. The high-affinity LTB 4 receptor, BLT1 is predominantly expressed on peripheral blood leukocytes and is known to modulate many chronic inflammatory diseases such as arthritis, atherosclerosis, allergic inflammation and insulin resistance during diet-induced obesity [17] , [18] , [19] , [20] . In this study, using the K-ras LA1 mice that develop spontaneous lung tumours [21] , we sought to establish a link between CS-induced chronic inflammation and lung tumour progression. CS exposure led to increased incidence of lung tumours and this process was attenuated in the absence of BLT1. The CS-induced pulmonary inflammation and, in particular, neutrophil recruitment were abrogated in BLT1 −/− mice. Furthermore, CS exposure enhanced the growth of implantable lung tumours leading to reduced survival. Since neutrophils are known to promote lung cancer [22] , [23] , we investigated the cellular and molecular mechanisms involved in CS-mediated neutrophil recruitment to lungs. The results suggest an intricate interplay of mast cell-, macrophage- and epithelial cell-derived lipid chemoattractant (LTB 4 ), cytokine (interleukin (IL)-1β) and neutrophil-active chemokines in coordinating CS-induced neutrophil migration. BLT1-mediated recruitment of neutrophils through mast cell-produced LTB 4 appears to be the critical initial event in promoting CS-induced inflammation. Collectively, our findings suggest potential for targeting BLT1-mediated neutrophil recruitment for combating silicosis and associated lung cancer. Absence of BLT1 abrogates the CS-promoted lung tumour growth Spontaneous activation of K-ras induces an inflammatory microenvironment that promotes tumour growth [24] . To investigate the involvement of BLT1-mediated inflammation in spontaneous K-ras activation-induced lung tumour progression, BLT1 −/− K-ras LA1 mice were generated. We found that the K-ras LA1 mice showed distinctly visible lung tumours at the age of 105 days, whereas the BLT1 −/− K-ras LA1 mice showed fewer and smaller tumours ( Supplementary Fig. 1a ). Detailed histopathological analysis of lungs performed after serial sectioning of the entire lungs at 200-μm intervals showed that both BLT1 +/+ K-ras LA1 and BLT1 −/− K-ras LA1 mice developed similar lung lesions ( Supplementary Fig. 1b ). However, the numbers of such lesions were significantly reduced in BLT1 −/− K-ras LA1 mice ( Supplementary Fig. 1c ). To examine the effect of CS exposure on lung tumour growth, K-ras LA1 mice were instilled with CS. To determine the role of BLT1-mediated inflammation in this process, BLT1 −/− K-ras LA1 mice were also exposed to CS. Equivalent exposure of CS in the lungs of both groups of mice was observed ( Fig. 1a,b ) and tumours were scored in the histological sections. Following CS exposure, the BLT1 +/+ K-ras LA1 mice exhibited a significant increase in lung adenomas, the most common histological type found in 100% of each cohort ( Fig. 1c,d ). In contrast, complete attenuation of increase in lung tumour incidence was observed in CS-exposed BLT1 −/− K-ras LA1 mice. These data suggest that CS exposure accelerates lung tumour growth through a process that requires BLT1. 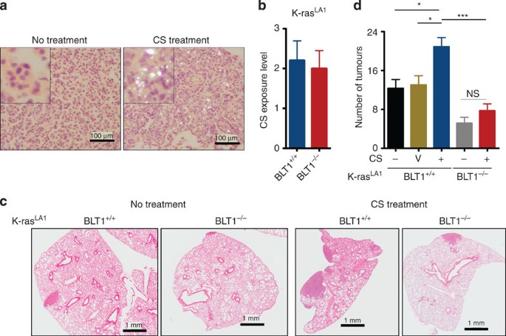Figure 1: CS-promoted lung tumour progression is abrogated in the absence of BLT1. Forty-five-day-old BLT1+/+K-rasLA1and BLT1−/−K-rasLA1mice were exposed to CS by intra-tracheal instillation as described in methods. Sixty days post CS instillation, lungs from these mice were analysed for CS particle deposition and tumour multiplicity. (a) Representative lung haematoxylin and eosin sections showing deposited CS particles; scale bars, 100 μm; insets show CS particles at higher magnification. (b) Lung CS exposure was determined based on semi-quantitative scoring (scale of 0–3) of CS particle deposition in sections;n=5 for both groups. (c) Representative lung lobe sections showing adenomas; scale bars, 1 mm. (d) Quantification of adenomas from all serial lung sections of different groups of animals and treatments as indicated; V indicates vehicle (PBS)-alone treatment. The number of mice in each group are: untreated BLT1+/+K-rasLA1(n=7); PBS-treated BLT1+/+K-rasLA1(n=5); CS-treated BLT1+/+K-rasLA1(n=10); untreated BLT1−/−K-rasLA1(n=7); CS-treated BLT1−/−K-rasLA1(n=10). Error bars inbandddenote mean±s.e.m. *P<0.025, ***P<0.0003, NS is not significant; Mann–WhitneyU-test. Figure 1: CS-promoted lung tumour progression is abrogated in the absence of BLT1. Forty-five-day-old BLT1 +/+ K-ras LA1 and BLT1 −/− K-ras LA1 mice were exposed to CS by intra-tracheal instillation as described in methods. Sixty days post CS instillation, lungs from these mice were analysed for CS particle deposition and tumour multiplicity. ( a ) Representative lung haematoxylin and eosin sections showing deposited CS particles; scale bars, 100 μm; insets show CS particles at higher magnification. ( b ) Lung CS exposure was determined based on semi-quantitative scoring (scale of 0–3) of CS particle deposition in sections; n =5 for both groups. ( c ) Representative lung lobe sections showing adenomas; scale bars, 1 mm. ( d ) Quantification of adenomas from all serial lung sections of different groups of animals and treatments as indicated; V indicates vehicle (PBS)-alone treatment. The number of mice in each group are: untreated BLT1 +/+ K-ras LA1 ( n =7); PBS-treated BLT1 +/+ K-ras LA1 ( n =5); CS-treated BLT1 +/+ K-ras LA1 ( n =10); untreated BLT1 −/− K-ras LA1 ( n =7); CS-treated BLT1 −/− K-ras LA1 ( n =10). Error bars in b and d denote mean±s.e.m. * P <0.025, *** P <0.0003, NS is not significant; Mann–Whitney U -test. Full size image BLT1 controls CS-induced pulmonary neutrophil recruitment We speculated that CS-mediated increase in lung tumour incidence may be related to increased inflammation, an essential feature of silicosis. A close association of chronic inflammation and tumour promotion has been observed in various types of cancers [1] , [25] . Therefore, we investigated the role of BLT1 in regulating CS-mediated chronic inflammation and thus controlling the pace of tumour growth. Histopathological examination of lung sections was carried out to assess inflammation. Features of acute silicosis including neutrophil aggregates, organizing pneumonia, type II pneumocyte proliferation, oedema and fibroblastic proliferation, as well as chronic inflammation features such as lymphocytic aggregates and expansion of interalveolar septa were all observed at 60 days post CS exposure in BLT1 +/+ K-ras LA1 mice ( Fig. 2a ). Although CS-exposed BLT1 −/− K-ras LA1 mice lungs also showed these histological features, the overall inflammation was significantly reduced in these mice ( Fig. 2a,b ). In independent cohorts of CS-treated BLT1 +/+ K-ras LA1 mice, analysis of bronchoalveolar lavage fluids (BALFs) 60 days post CS exposure by flow cytometry showed a significant increase in different leukocyte populations including neutrophils, macrophages and lymphocytes ( Fig. 2c ). Similar increases in macrophages and lymphocytes were also seen in CS-exposed BLT1 −/− K-ras LA1 mice, but the neutrophil numbers were significantly lower compared with CS-exposed BLT1 +/+ K-ras LA1 mice ( Fig. 2c ). Immunohistochemical analysis also showed similar levels of macrophage infiltration into lungs of both BLT1 +/+ K-ras LA1 and BLT1 −/− K-ras LA1 mice ( Supplementary Fig. 2 ). 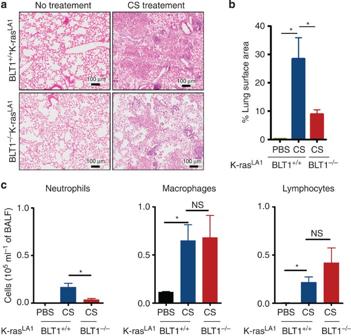Figure 2: Absence of BLT1 attenuates lung inflammation in K-rasLA1mice. Lungs from BLT1+/+K-rasLA1and BLT1−/−K-rasLA1mice exposed to CS for 60 days were assessed for inflammation and inflammatory cell recruitment. (a) Representative lung haematoxylin and eosin (H&E) sections show inflammation post CS treatment; scale bars, 100 μm. (b) Lung inflammation was scored as the percentage of inflamed lung area to total lung area in H&E-stained lung sections. The number of mice in each group are: PBS-treated BLT1+/+K-rasLA1(n=3); CS-treated BLT1+/+K-rasLA1(n=8); CS-treated BLT1−/−K-rasLA1(n=10). (c) CS-exposure-induced recruitment of neutrophils, macrophages and lymphocytes into airways was assessed in whole-lung lavage by flow cytometry as described in methods. The number of mice in each group are: PBS-treated BLT1+/+K-rasLA1(n=3); CS-treated BLT1+/+K-rasLA1(n=4); CS-treated BLT1−/−K-rasLA1(n=5). Error bars inbandcdenote mean±s.e.m. *P<0.04 Mann–WhitneyU-test. Figure 2: Absence of BLT1 attenuates lung inflammation in K-ras LA1 mice. Lungs from BLT1 +/+ K-ras LA1 and BLT1 −/− K-ras LA1 mice exposed to CS for 60 days were assessed for inflammation and inflammatory cell recruitment. ( a ) Representative lung haematoxylin and eosin (H&E) sections show inflammation post CS treatment; scale bars, 100 μm. ( b ) Lung inflammation was scored as the percentage of inflamed lung area to total lung area in H&E-stained lung sections. The number of mice in each group are: PBS-treated BLT1 +/+ K-ras LA1 ( n =3); CS-treated BLT1 +/+ K-ras LA1 ( n =8); CS-treated BLT1 −/− K-ras LA1 ( n =10). ( c ) CS-exposure-induced recruitment of neutrophils, macrophages and lymphocytes into airways was assessed in whole-lung lavage by flow cytometry as described in methods. The number of mice in each group are: PBS-treated BLT1 +/+ K-ras LA1 ( n =3); CS-treated BLT1 +/+ K-ras LA1 ( n =4); CS-treated BLT1 −/− K-ras LA1 ( n =5). Error bars in b and c denote mean±s.e.m. * P <0.04 Mann–Whitney U -test. Full size image Since activated K-ras mutations are known to activate an intrinsic pathway of inflammation, we also analysed CS-induced inflammation in BLT1 +/+ and BLT1 −/− mice. Significant influx of leukocytes into the airways was observed in these mice ( Fig. 3a,c ). In airways, neutrophil influx peaked very early at day 2, decreased by day 6 and again increased by day 30. However, neutrophil influx was significantly attenuated during the acute phase at day 2 and the chronic phase at day 30 in BLT1 −/− mice ( Fig. 3b,c ). In contrast, macrophage and lymphocyte influx was found to be similar in both BLT1 +/+ and BLT1 −/− mice at 2, 6 or 30 days post CS exposure. To determine whether cellular distribution in the airways reflected changes in the total lungs, whole-lung digests were analysed by flow cytometry. At 2 days post CS exposure, there was an increase in neutrophil influx in BLT1 +/+ mice that was significantly reduced in BLT1 −/− mice ( Fig. 3d ). 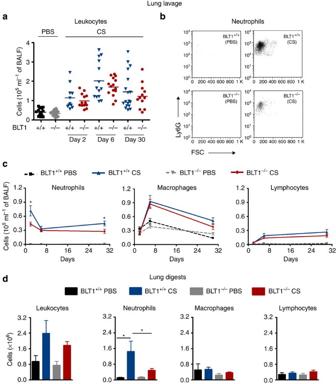Figure 3: Attenuation of CS-induced lung neutrophil recruitment in the absence of BLT1. Eight-week-old BLT1+/+and BLT1−/−mice were exposed to CS. Inflammatory cell recruitment into airways (a–c) and lung interstitium (d) was assessed by flow cytometry using surface staining for cell-specific markers. Analysis of whole-lung lavage at indicated times show (a) number of total leukocytes; each dot represents a single mouse, (b) neutrophils 2 days post CS exposure in the flow cytometry scatter plots and (c) number of neutrophils, macrophages and lymphocytes. Data represent at least 11 mice per group; difference between CS-treated BLT1+/+and BLT1−/−group is indicated. (d) Analysis of unlavaged whole-lung digests 2 days post CS exposure show number of total leukocytes, neutrophils, macrophages and lymphocytes. The number of mice in each group are: PBS-treated BLT1+/+(n=3); CS-treated BLT1+/+(n=5); PBS-treated BLT1−/−(n=5); CS-treated BLT1−/−(n=6). Error bars denote mean±s.e.m. *P<0.04 Mann–WhitneyU-test. Figure 3: Attenuation of CS-induced lung neutrophil recruitment in the absence of BLT1. Eight-week-old BLT1 +/+ and BLT1 −/− mice were exposed to CS. Inflammatory cell recruitment into airways ( a – c ) and lung interstitium ( d ) was assessed by flow cytometry using surface staining for cell-specific markers. Analysis of whole-lung lavage at indicated times show ( a ) number of total leukocytes; each dot represents a single mouse, ( b ) neutrophils 2 days post CS exposure in the flow cytometry scatter plots and ( c ) number of neutrophils, macrophages and lymphocytes. Data represent at least 11 mice per group; difference between CS-treated BLT1 +/+ and BLT1 −/− group is indicated. ( d ) Analysis of unlavaged whole-lung digests 2 days post CS exposure show number of total leukocytes, neutrophils, macrophages and lymphocytes. The number of mice in each group are: PBS-treated BLT1 +/+ ( n =3); CS-treated BLT1 +/+ ( n =5); PBS-treated BLT1 −/− ( n =5); CS-treated BLT1 −/− ( n =6). Error bars denote mean±s.e.m. * P <0.04 Mann–Whitney U -test. Full size image Absence of BLT1 does not impair CS-induced chemokine production Since absence of BLT1 was found to attenuate neutrophil recruitment to lungs, we sought to analyze whether deletion of BLT1 had an effect on the production of cytokines and chemokines involved in CS-induced neutrophilic inflammation. Levels of the BLT1 ligand LTB 4 were found to significantly increase in BALFs of BLT1 +/+ mice at 2, 6 or 30 days post CS exposure ( Fig. 4a ). A significant increase in LTB 4 was also observed in BLT1 +/+ K-ras LA1 mice ( Fig. 4b ) 60 days post CS exposure. In BLT1 −/− mice, similar increase in LTB 4 levels was observed at all tested time points, with the exception of day 2 ( Fig. 4a,b ). 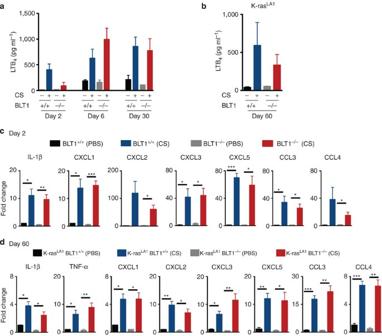Figure 4: CS-induced neutrophil chemoattractants remain unaffected in the absence of BLT1. Mediators of CS-induced pulmonary inflammation were analysed by accessing production of (a,b) LTB4in whole-lung lavage fluids and (c,d) cytokines and chemokines in total lung RNA. LTB4levels in lung lavage fluids of (a) CS-exposed BLT1+/+and BLT1−/−mice at indicated times and (b) of BLT1+/+K-rasLA1and BLT1−/−K-rasLA1mice exposed to CS for 60 days. Data are from at least five mice per group. Quantitative real-time PCR analysis of total lung RNA showing fold increase of neutrophil-active cytokines and chemokines in (c) BLT1+/+and BLT1−/−mice exposed to CS for 2 days and (d) BLT1+/+K-rasLA1and BLT1−/−K-rasLA1mice exposed to CS for 60 days. Fold change of messenger RNA (mRNA) levels over PBS-treated BLT1+/+samples are shown; differences in mRNA levels are not significant between the CS-exposed BLT1+/+and BLT1−/−groups. Data represent at least five mice per group; error bars denote mean±s.e.m. *P<0.03, **P<0.009, ***P<0.0007; unpairedt-test. Figure 4: CS-induced neutrophil chemoattractants remain unaffected in the absence of BLT1. Mediators of CS-induced pulmonary inflammation were analysed by accessing production of ( a , b ) LTB 4 in whole-lung lavage fluids and ( c , d ) cytokines and chemokines in total lung RNA. LTB 4 levels in lung lavage fluids of ( a ) CS-exposed BLT1 +/+ and BLT1 −/− mice at indicated times and ( b ) of BLT1 +/+ K-ras LA1 and BLT1 −/− K-ras LA1 mice exposed to CS for 60 days. Data are from at least five mice per group. Quantitative real-time PCR analysis of total lung RNA showing fold increase of neutrophil-active cytokines and chemokines in ( c ) BLT1 +/+ and BLT1 −/− mice exposed to CS for 2 days and ( d ) BLT1 +/+ K-ras LA1 and BLT1 −/− K-ras LA1 mice exposed to CS for 60 days. Fold change of messenger RNA (mRNA) levels over PBS-treated BLT1 +/+ samples are shown; differences in mRNA levels are not significant between the CS-exposed BLT1 +/+ and BLT1 −/− groups. Data represent at least five mice per group; error bars denote mean±s.e.m. * P <0.03, ** P <0.009, *** P <0.0007; unpaired t -test. Full size image To determine global changes in CS-induced gene expression profiles, total RNA isolated from lungs was analysed by microarrays. The data analysis indicated that several markers and mediators of inflammation increased in BLT1 +/+ and BLT1 −/− mice at 2 days post CS exposure, as well as in BLT1 +/+ K-ras LA1 and BLT1 −/− K-ras LA1 mice at 60 days post CS exposure. Of interest, inflammatory cytokines such as IL-1β and tumour necrosis factor (TNF)-α, as well as number of chemokines and their receptors were upregulated upon CS exposure ( Supplementary Fig. 3 ). Real-time PCR analysis confirmed the CS-induced increase in neutrophil-active cytokines and chemokines both at early (day 2) and late (day 60) times, both in the presence and absence of BLT1 ( Fig. 4c,d ). Multiplex analysis of neutrophil-active chemokines in BALFs also showed significant increase upon CS exposure, both in the presence and absence of BLT1 ( Supplementary Fig. 4 ). This suggests that neutrophil-active cytokines and chemokines may be produced in the absence of BLT1 signalling and yet are not sufficient to overcome attenuation of neutrophil influx in BLT1 −/− lungs. Cellular mediators of CS-induced inflammation In inflamed lungs, neutrophil-active cytokines and chemokines may be produced from lung resident cells or recruited leukocytes. We next analysed the CS-induced production of LTB 4 , IL-1β and neutrophil-active chemokines in vitro by the lung adenocarcinoma cell line derived from K-ras LA1 mice-LKR13 (ref. 24 ) and various murine primary cells including macrophages, neutrophils, mast cells and splenocytes. Among the primary cells, macrophages and neutrophils, but not splenocytes, produced LTB 4 upon CS exposure ( Fig. 5a ). Bone-marrow-derived mast cells (BMMCs) produced the highest levels of CS-induced LTB 4 in a dose-dependent manner that peaked by 3 h ( Fig. 5a ; Supplementary Fig. 5a,b ). CS-activated murine macrophages produced IL-1β, whereas mast cells and splenocytes did not secrete IL-1β ( Fig. 5b ). Primary macrophages and mast cells isolated from murine lungs were also tested for their ability to produce LTB 4 and IL-1β. CS activation of alveolar macrophages led to production of both LTB 4 and IL-1β, whereas lung mast cells produced LTB 4 but not IL-1β post CS exposure ( Fig. 5c,d ). 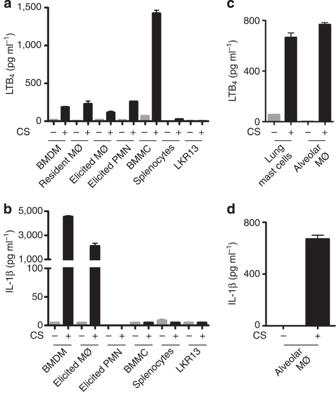Figure 5: Cell type specificity of CS-induced LTB4and IL-1β production. Lung epithelial cell line (LKR13) and primary cells: macrophages, mast cells, neutrophils and splenocytes from wild-type (WT) were assessed for production of LTB4and IL-1βin vitropost CS stimulation. In triplicate cultures, 0.3 × 106of the indicated cell types were stimulated with 100 μg cm−2of CS for 6 h. (a) LTB4levels in culture supernatants of CS-exposedex vivocultured immune cells and lung epithelial cell line (LKR13) as indicated; MØ is macrophage, PMN is neutrophil, BMDM is bone-marrow-derived macrophages and BMMC is bone-marrow-derived mast cells. (b) IL-1β levels in the same culture supernatants as ina. The CS-induced LTB4(c) and IL-1β (d) production was determined in culture supernatants of alveolar macrophages and lung mast cells. Alveolar macrophages and lung mast cells were purified as described in methods and exposed to CSin vitro. Purity of the cell types was determined by flow cytometry. Thioglycollate-elicited neutrophils and macrophages, resident peritoneal macrophages and lung mast cells were ≥95% pure, whereas BMMC, BMDM and alveolar macrophages were ≥99% pure. Error bars denote mean±s.e.m. Data are representative of at least two independent experiments in triplicate cultures. Figure 5: Cell type specificity of CS-induced LTB 4 and IL-1β production. Lung epithelial cell line (LKR13) and primary cells: macrophages, mast cells, neutrophils and splenocytes from wild-type (WT) were assessed for production of LTB 4 and IL-1β in vitro post CS stimulation. In triplicate cultures, 0.3 × 10 6 of the indicated cell types were stimulated with 100 μg cm −2 of CS for 6 h. ( a ) LTB 4 levels in culture supernatants of CS-exposed ex vivo cultured immune cells and lung epithelial cell line (LKR13) as indicated; MØ is macrophage, PMN is neutrophil, BMDM is bone-marrow-derived macrophages and BMMC is bone-marrow-derived mast cells. ( b ) IL-1β levels in the same culture supernatants as in a . The CS-induced LTB 4 ( c ) and IL-1β ( d ) production was determined in culture supernatants of alveolar macrophages and lung mast cells. Alveolar macrophages and lung mast cells were purified as described in methods and exposed to CS in vitro . Purity of the cell types was determined by flow cytometry. Thioglycollate-elicited neutrophils and macrophages, resident peritoneal macrophages and lung mast cells were ≥95% pure, whereas BMMC, BMDM and alveolar macrophages were ≥99% pure. Error bars denote mean±s.e.m. Data are representative of at least two independent experiments in triplicate cultures. Full size image The LTB 4 production by CS activation in the macrophage cell-line RAW264.7 was completely blocked by 5-lipoxygenase (5-LO) inhibitor, Zileuton ( Supplementary Fig. 6a–c ). The CS-induced LTB 4 was biologically active as determined by chemotaxis of 300.19 cells expressing BLT1 as well as BLT1 +/+ neutrophils but not the parental 300.19 cells or BLT1 −/− neutrophils ( Supplementary Fig. 6d,e ). Independent regulation of CS-induced LTB 4 and IL-1-β production Since both LTB 4 and IL-1β appear to be critical for silicosis, the interdependence of their production was analysed. CS-exposed mast cells from inflammasome pathway-deficient (NALP3 −/− , ASC −/− and IL-1αβ −/− ) or IL-1 response-deficient mice (IL-1R −/− , MyD88 −/− ), as well as BLT1 −/− mice, secreted LTB 4 , but not the 5-LO −/− mast cells ( Fig. 6a ). As expected, CS-treated macrophages from inflammasome pathway-deficient (NALP3 −/− , ASC −/− and IL-1αβ −/− ) mice did not secrete IL-1β, while macrophages from 5-LO pathway-deficient (BLT1 −/− or 5-LO −/− ) mice were found to secrete IL-1β similar to wild-type (WT) macrophages ( Fig. 6b ). These data suggest that CS-induced activation of 5-LO and the inflammasome pathway are completely independent of each other, and absence of BLT1 does not affect either of the pathways. 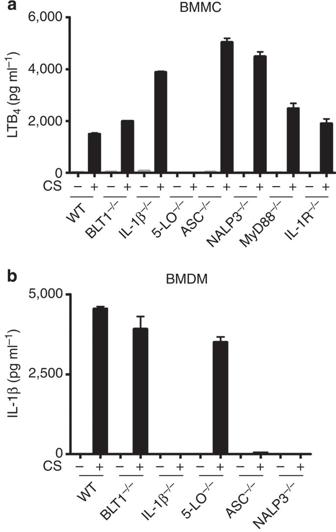Figure 6: Independent regulation of LTB4and IL-1β production in CS-exposed cells. Interdependence of CS-induced LTB4and IL-1β production was determined in cultured bone-marrow-derived mast cells (BMMCs) and bone-marrow-derived macrophages (BMDMs) from different gene knockout mice as indicated. In triplicate cultures, 0.3 × 106of (a) BMMCs or (b) BMDMs were stimulated with 100 μg cm−2of CS for 6 h and (a) LTB4and (b) IL-1β levels were determined by the enzyme immunoassay or enzyme-linked immunosorbent assay, respectively. Purity of the cells was determined by flow cytometry. All cell types of indicated genotypes were ≥99% pure. Error bars denote mean±s.e.m. Data are representative of at least two independent experiments performed in triplicate cultures. Figure 6: Independent regulation of LTB 4 and IL-1β production in CS-exposed cells. Interdependence of CS-induced LTB 4 and IL-1β production was determined in cultured bone-marrow-derived mast cells (BMMCs) and bone-marrow-derived macrophages (BMDMs) from different gene knockout mice as indicated. In triplicate cultures, 0.3 × 10 6 of ( a ) BMMCs or ( b ) BMDMs were stimulated with 100 μg cm −2 of CS for 6 h and ( a ) LTB 4 and ( b ) IL-1β levels were determined by the enzyme immunoassay or enzyme-linked immunosorbent assay, respectively. Purity of the cells was determined by flow cytometry. All cell types of indicated genotypes were ≥99% pure. Error bars denote mean±s.e.m. Data are representative of at least two independent experiments performed in triplicate cultures. Full size image Although LKR13 cells did not secrete LTB 4 or IL-1β ( Fig. 5a,b ), they produced neutrophil-active chemokines CXCL1, CXCL2, CXCL3, CXCL5 and CCL5 in response to CS stimulation, suggesting that pathways leading to the production of these chemokines are most likely independent of 5-LO or inflammasome activation ( Supplementary Fig. 7 ). Many of these chemokines were also produced by both BLT1 +/+ and BLT1 −/− macrophages and mast cells ( Supplementary Fig. 7 ). CS-induced inflammation in an air-pouch model requires BLT1 The in vitro studies showed that mast cells are a major source of LTB 4 production, and the absence of BLT1 clearly reduced lung inflammation and neutrophil influx in vivo . Previous studies have shown that CS-mediated lung inflammation is dependent on the presence of mast cells [26] . We adopted the murine air-pouch model [27] to assess the contribution of mast cells and the role of the LTB 4 –BLT1 axis in neutrophil recruitment during CS-induced inflammation. In this model, CS exposure of BLT1 +/+ mice induced the production of LTB 4 ( Fig. 7a ) accompanied by influx of neutrophils ( Fig. 7b,c ). This response, however, was significantly dampened in the BLT1 −/− as well as in mast cell-deficient mice ( Fig. 7a–c ). These data show that neutrophil recruitment is an early event during CS exposure and is controlled by mast cell-mediated LTB 4 production and expression of BLT1 on neutrophils. 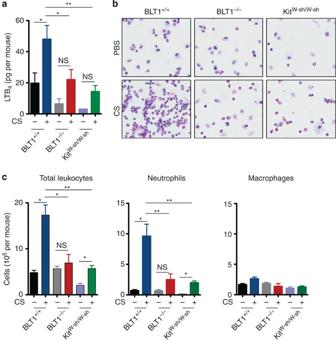Figure 7: CS-induced neutrophil recruitment into the air pouch is dependent on the LTB4/BLT1 axis. CS-induced inflammation in an air pouch was analysed. Six hours post CS particle exposure, the air pouch was lavaged with 3 ml of buffer to assess LTB4levels and infiltrating immune cells. (a) LTB4levels, (b) leukocytes on cytospin slides and (c) total leukocytes, neutrophils and macrophages as identified by flow cytometry of the air-pouch lavage fluid from mice of the indicated genotypes. Data are representative of at least five mice per group. Error bars denote mean±s.e.m. *P<0.02, **P<0.009; NS, not significant; Mann–WhitneyU-test. Figure 7: CS-induced neutrophil recruitment into the air pouch is dependent on the LTB 4 /BLT1 axis. CS-induced inflammation in an air pouch was analysed. Six hours post CS particle exposure, the air pouch was lavaged with 3 ml of buffer to assess LTB 4 levels and infiltrating immune cells. ( a ) LTB 4 levels, ( b ) leukocytes on cytospin slides and ( c ) total leukocytes, neutrophils and macrophages as identified by flow cytometry of the air-pouch lavage fluid from mice of the indicated genotypes. Data are representative of at least five mice per group. Error bars denote mean±s.e.m. * P <0.02, ** P <0.009; NS, not significant; Mann–Whitney U -test. Full size image CS-induced inflammation promotes implanted lung tumour To determine whether CS accelerates the growth of implanted lung tumours, we adopted LKR13 subcutaneous (s.c.) tumour model. LKR13 cells mixed with CS particles in matrigel were implanted s.c. into Rag2 −/− mice. In BLT1 +/+ Rag2 −/− mice, CS exposure led to a significant increase in tumour growth and consequently reduced their survival ( Fig. 8a–d ). Interestingly, the BLT1 −/− Rag2 −/− mice displayed reduced tumour growth and survival advantage ( Fig. 8a–d ). Analysis of immune cell infiltration in these tumours showed that presence of CS resulted in increased neutrophil influx, whereas macrophages and mast cells remained unchanged in BLT1 +/+ Rag2 −/− mice ( Fig. 8e ). In tumours growing in BLT1 −/− Rag2 −/− mice, neutrophil influx was significantly reduced compared with BLT1 +/+ Rag2 −/− mice, whereas the macrophage and mast cell numbers were unchanged. Analysis of neutrophil-active chemokines indicated significant attenuation in the levels of LTB 4 , CXCL1 and CCL3 in BLT1 −/− mice post CS exposure ( Fig. 8e,f ). These results emphasize a direct role for CS in promoting lung tumour growth that is dependent on LTB 4 /BLT1-mediated inflammation. 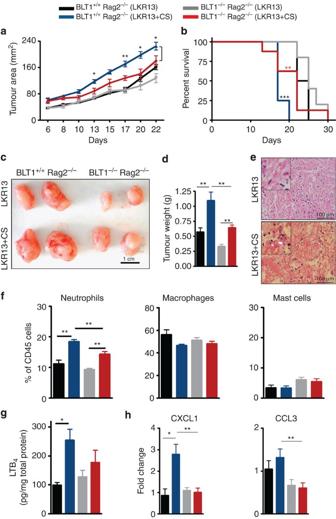Figure 8: Absence of BLT1 protects from CS-promoted growth of implanted lung tumours. LKR13 cells along with CS particles were implanted subcutaneously into BLT1+/+Rag2−/−or BLT1−/−Rag2−/−mice and the kinetics of tumour growth, survival of mice and tumour inflammatory microenvironment was analysed. (a) Tumour size in mice of indicated genotype and treatment are shown. The number of mice in each group are: LKR13-injected BLT1+/+Rag2−/−(n=12); LKR13 with CS-injected BLT1+/+Rag2−/−(n=10); LKR13-injected BLT1−/−Rag2−/−(n=6); LKR13 with CS-injected BLT1−/−Rag2−/−(n=7). (b) Kaplan–Meier survival curves of tumour-bearing mice are shown. Data represent eight mice per group; *** (black) indicates comparison between LKR13 and LKR13 with CS-injected BLT1+/+Rag2−/−groups; ** (red) indicates comparison between LKR13 with CS-injected BLT1+/+Rag2−/−and BLT1−/−Rag2−/−groups. (c) Representative images of tumours 16 days post implantation for the indicated genotype and treatment are shown; scale bars, 1 cm. (d) Tumour weights at day 16 of LKR13-injected BLT1+/+Rag2−/−(n=4); LKR13 with CS-injected BLT1+/+Rag2−/−(n=6); LKR13-injected BLT1−/−Rag2−/−(n=5); LKR13 with CS-injected BLT1−/−Rag2−/−(n=7). (e) Deposited CS particles in tumour sections viewed under polarized light; scale bars, 100 μm; insets show CS particles at higher magnification. (f) Neutrophils, macrophages and mast cells expressed as percent of total tumour-infiltrating immune cells identified by flow cytometry are shown. (g) LTB4levels measured in tumour homogenates and (h) quantitative real-time PCR analysis of total tumour RNA showing fold increase of neutrophil-active chemokines; fold change over BLT1+/+Rag2−/−injected with LKR13 cells is shown. Inf–h, the number of mice in each group are: LKR13-injected BLT1+/+Rag2−/−(n=4), LKR13-injected BLT1−/−Rag2−/−(n=4), LKR13 with CS-injected BLT1+/+Rag2−/−(n=7) and LKR13 with CS-injected BLT1−/−Rag2−/−(n=7). Error bars denote mean±s.e.m. *P<0.02, **P<0.009, ***P<0.0007; Mann–WhitneyU-test. Figure 8: Absence of BLT1 protects from CS-promoted growth of implanted lung tumours. LKR13 cells along with CS particles were implanted subcutaneously into BLT1 +/+ Rag2 −/− or BLT1 −/− Rag2 −/− mice and the kinetics of tumour growth, survival of mice and tumour inflammatory microenvironment was analysed. ( a ) Tumour size in mice of indicated genotype and treatment are shown. The number of mice in each group are: LKR13-injected BLT1 +/+ Rag2 −/− ( n =12); LKR13 with CS-injected BLT1 +/+ Rag2 −/− ( n =10); LKR13-injected BLT1 −/− Rag2 −/− ( n =6); LKR13 with CS-injected BLT1 −/− Rag2 −/− ( n =7). ( b ) Kaplan–Meier survival curves of tumour-bearing mice are shown. Data represent eight mice per group; *** (black) indicates comparison between LKR13 and LKR13 with CS-injected BLT1 +/+ Rag2 −/− groups; ** (red) indicates comparison between LKR13 with CS-injected BLT1 +/+ Rag2 −/− and BLT1 −/− Rag2 −/− groups. ( c ) Representative images of tumours 16 days post implantation for the indicated genotype and treatment are shown; scale bars, 1 cm. ( d ) Tumour weights at day 16 of LKR13-injected BLT1 +/+ Rag2 −/− ( n =4); LKR13 with CS-injected BLT1 +/+ Rag2 −/− ( n =6); LKR13-injected BLT1 −/− Rag2 −/− ( n =5); LKR13 with CS-injected BLT1 −/− Rag2 −/− ( n =7). ( e ) Deposited CS particles in tumour sections viewed under polarized light; scale bars, 100 μm; insets show CS particles at higher magnification. ( f ) Neutrophils, macrophages and mast cells expressed as percent of total tumour-infiltrating immune cells identified by flow cytometry are shown. ( g ) LTB 4 levels measured in tumour homogenates and ( h ) quantitative real-time PCR analysis of total tumour RNA showing fold increase of neutrophil-active chemokines; fold change over BLT1 +/+ Rag2 −/− injected with LKR13 cells is shown. In f – h , the number of mice in each group are: LKR13-injected BLT1 +/+ Rag2 −/− ( n =4), LKR13-injected BLT1 −/− Rag2 −/− ( n =4), LKR13 with CS-injected BLT1 + / + Rag2 −/− ( n =7) and LKR13 with CS-injected BLT1 − / − Rag2 −/− ( n =7). Error bars denote mean±s.e.m. * P <0.02, ** P <0.009, *** P <0.0007; Mann–Whitney U -test. Full size image Exposure to CS has long been associated with increased susceptibility to lung cancer in humans [8] . The results presented here show that CS promotes tumour progression in well-defined spontaneous and implantable mouse lung tumour models. The data suggest that complex interplay of cellular and molecular mediators orchestrate CS-mediated lung inflammation. Mast cells and macrophages produce LTB 4 and IL-1β upon CS exposure, leading to sustained neutrophilic inflammation that is further maintained by the chemokines produced by the lung epithelial cells ( Fig. 9 ). This chronic inflammatory microenvironment promotes lung tumour progression. 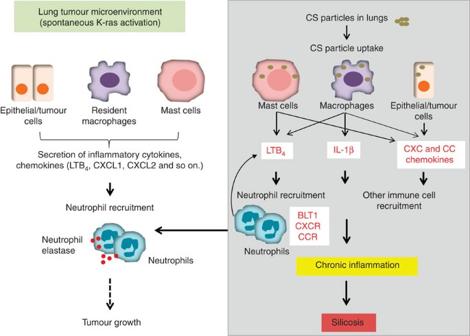Figure 9: A schematic model for the role of the LTB4–BLT1 axis in CS-accelerated lung tumour growth. Spontaneous activation of K-ras gene in the lungs induces an inflammatory microenvironment (intrinsic pathway) that promotes cancer-related inflammation and tumour growth. This study shows that exposure to crystalline silica particles induces chronic inflammation (extrinsic pathway), which likely accelerates lung tumour growth. LTB4produced by mast cells and IL1β, LTB4, CXC/CC chemokines by macrophages and CXC/CC chemokines by lung epithelial cells in response to CS exposure leads to sustained neutrophil accumulation. LTB4/BLT1 axis sets the pace of CS-induced sterile inflammation, thereby promoting lung tumour progression. Figure 9: A schematic model for the role of the LTB 4 –BLT1 axis in CS-accelerated lung tumour growth. Spontaneous activation of K-ras gene in the lungs induces an inflammatory microenvironment (intrinsic pathway) that promotes cancer-related inflammation and tumour growth. This study shows that exposure to crystalline silica particles induces chronic inflammation (extrinsic pathway), which likely accelerates lung tumour growth. LTB 4 produced by mast cells and IL1β, LTB 4 , CXC/CC chemokines by macrophages and CXC/CC chemokines by lung epithelial cells in response to CS exposure leads to sustained neutrophil accumulation. LTB 4 /BLT1 axis sets the pace of CS-induced sterile inflammation, thereby promoting lung tumour progression. Full size image Lung tumour progression is associated with activation of both intrinsic and extrinsic pathways of inflammation [1] , [2] , [7] . Transforming mutations in the K-ras oncogene found in ∼ 30% of human lung adenocarcinomas activate the intrinsic pathway of inflammation by activating NF-kB and consequent production of cytokines and chemokines [24] , [28] . Inflammation initiated by extrinsic factors such as exposure to CS may also promote cigarette smoke carcinogen-induced tumour progression [8] . While CS has been designated as a human carcinogen by IARC (International Agency for Research on Cancer) [8] , the causal relationship of CS exposure and lung cancer progression remained unclear due to lack of experimental model systems. Recent studies have shown that NNK (4-(N-methyl-N-nitrosamino)-1-(3-pyridyl)-1-butanone)-initiated lung tumour incidence is increased upon CS exposure [29] . In this study, we provide evidence that CS exposure accelerates lung tumour growth in a spontaneous K-ras LA1 mouse model ( Fig. 1 ) and this enhancement is dependent on BLT1-mediated chronic inflammation ( Fig. 2 ). Furthermore, the s.c implantable lung tumour model provided direct evidence for the tumour-promoting effects of CS ( Fig. 8 ). Co-implantation of K-ras-mutated lung tumour cells with CS resulted in accelerated tumour growth that reduced the survival of tumour-bearing mice. In this model also absence of BLT1 reduced the tumour burden and improved survival, suggesting that BLT1-mediated inflammation is a crucial component in CS-induced tumour promotion. CS exposure is known to induce cell death [30] , leading to the recruitment and activation of a variety of leukocytes including mast cells, macrophages and neutrophils. The data herein outline the cellular and molecular basis for CS-induced inflammation ( Fig. 9 ). Mast cells are known to be essential for the full development of CS-induced lung inflammation and silicosis [31] . Studies presented here with cultured mast cells showed that CS exposure leads to significantly more LTB 4 production by mast cells relative to other myeloid cells, suggesting that mast cell activation is likely an important step in CS-induced inflammation ( Fig. 5 ). This was further substantiated by the observation of attenuated LTB 4 levels and neutrophils in the CS-exposed air pouch of mast cell-deficient mice ( Fig. 7 ). Mast cell-produced LTB 4 along with macrophage-secreted LTB 4 and IL-1β coordinates with the epithelial cell-generated chemokines to orchestrate neutrophil migration into inflamed lungs. Although CS exposure also leads to lymphocytic infiltration into lungs, it is known that innate immune processes are sufficient to drive silicosis in the absence of lymphocytes [32] . Consistent with this finding, splenocytes did not produce LTB 4 or IL-1β in response to CS activation ( Fig. 5a,b ). Earlier studies have shown that various cytokines and chemokines such as IL-β, TNF-α, TGF-β, IL-6, IL-8, IL-17A, CCL2 and CCL3 mediate silicosis [33] , [34] , [35] , [36] , [37] . Among these mediators, production of IL-1β through inflammasome activation appears to be most critical for CS-induced lung inflammation [36] , [38] , [39] , [40] . Our study shows that production of LTB 4 is also critical for CS-induced lung inflammation ( Fig. 4a,b ). However, in CS-exposed lungs absence of BLT1 did not influence production of mediators including IL-1β at early or late times in presence or absence of an activating K-ras mutation in vivo ( Fig. 4 ). Similarly, BLT1 deficiency also did not impact the production of IL-1β or neutrophil-active chemokines by CS-exposed cells in vitro ( Fig. 6b ; Supplementary Fig. 7 ). Moreover, CS exposure of the inflammasome pathway-deficient or IL-1-deficient mast cells did not impact the LTB 4 production ( Fig. 6a ). Thus, CS activates parallel pathways for the production of IL-1β and LTB 4 . Although neutrophil recruitment was significantly compromised in the absence of BLT1, it was not completely attenuated ( Figs 2c , 3c , 7c and 8c ) possibly due to the production of IL-1β and CC/CXC neutrophil chemokines. In various inflammatory diseases, relay of molecules that orchestrate recruitment of different cell types are of critical importance towards disease manifestation. In this regard, extremely coordinated tissue chemotaxis of neutrophils in mouse models of inflammatory arthritis [20] or sterile injury [41] were also shown to be initiated by LTB 4 . In arthritis models LTB 4 /BLT1 axis was critical for initial neutrophil recruitment into the joint, leading to the sequential production of IL-1β and neutrophil-active chemokine production that sustains joint inflammation. In contrast to these observations, current data show that absence of BLT1 did not impair production of neutrophil-active cytokine and chemokines in the CS-exposed lungs. A reduction in LTB 4 levels observed in the air pouch of BLT1 −/− mice were possibly due to impairment in recruitment of LTB 4 -producing neutrophils ( Fig. 7a ). Together, these data suggest that CS-exposed mast cells, macrophages and epithelial cells secrete lipids (LTB 4 )–cytokines (IL-1β)–chemokines (CXCL, CCL) independently of each other that coordinate recruitment of neutrophils. However, the LTB 4 –BLT1 axis plays the most critical role such that absence of BLT1 significantly dampens this response. Pro-tumorigenic activity of tumour-associated neutrophils is increasingly being appreciated in lung and other cancers [23] , [42] , [43] , [44] , [45] . Inhibition of CXCR2-mediated neutrophil infiltration into lung tumours was shown to be associated with reduced tumour growth [23] , [28] , [46] . Neutrophil numbers within the tumour correlates to poor prognosis in NSCLC [47] . Interestingly, in NSCLC patients an increase of neutrophil chemoattractants LTB 4 and IL-8 in exhaled breath condensate were reported [48] . Again, levels of LTB 4 and IL-8 were found to increase with progression of NSCLC stages I through IV, indicating the importance of LTB 4 and IL-8 in recruiting neutrophils into lung tumours. Thus, a common feature of lung cancer progression appears to be association of neutrophils in the tumour. The results presented here show a strong correlation between rapid tumour growth and increased neutrophilic inflammation and rapid tumour growth both in spontaneous and implantable lung tumour models. Furthermore, neutrophil recruitment is dependent on BLT1 expression under different settings including the lungs of K-ras LA1 mice, skin air pouch and in the s.c. implantable tumour models, suggesting a critical function for LTB 4 /BLT1 axis in regulating CS-mediated inflammation. While the neutrophilic inflammation is the most likely mediator of CS-promoted tumour progression, further studies are required to establish a direct cause and effect relationship in these models. Mice All mice were on C57BL/6 background and were sex and age matched at 6–7 weeks. K-ras LA1 mice were obtained from the NCI mouse repository and subsequently crossed onto BLT1 −/− background to generate BLT1 −/− K-ras LA1 mice. Rag2 −/− mice were obtained from Taconic (Germantown, NY) and subsequently crossed onto BLT1 −/− background to generate BLT1 −/− Rag2 −/− mice. C57BL/6J (BLT1 +/+ ), Kit W−sh/W−sh , MyD88 −/− mice were purchased from Jackson Laboratories. BLT1 −/− mice were described previously [49] . IL-1αβ −/− and 5-LO −/− mice were from Dr A. Luster. IL-1R −/− mice were kindly provided by Dr Jun Yan at the University of Louisville. Bone marrow from NALP3 −/− and ASC −/− mice were provided by Dr Kate Fitzgerald at the University of Massachusetts. All mice were maintained under specific pathogen-free conditions, and all the procedures were approved by University of Louisville Institutional Animal Care and Use Committee. CS instillation in mouse lungs CS (MIN-U-SIL-5; average particle diameter 1.7 μm) was obtained from US Silica Co., WV, and was made endotoxin-free by baking at 200 °C overnight. Forty-five-day-old BLT1 +/+ , BLT1 −/− , BLT1 +/+ K-ras LA1 and BLT1 −/− K-ras LA1 mice were either left untreated or surgically instilled (intra-tracheal) with endotoxin-free PBS (vehicle) or 2 mg of endotoxin-free CS suspended in vehicle without sonication. CS particle suspension was vortexed before instillation to avoid settling of the particles. Mice were treated with antibiotics for a week before surgery and were continuously maintained on antibiotics until euthanized. Lungs from BLT1 +/+ K-ras LA1 and BLT1 −/− K-ras LA1 mice were analysed 60 days after PBS or CS instillation and lungs from BLT1 +/+ , BLT1 −/− mice were analysed after 2, 6 or 30 days after PBS or CS instillation as indicated. CS-induced inflammation in the air-pouch model Six- to eight-week-old mice were used to generate an air pouch as described previously [50] . Briefly, mice were injected s.c. with 5 ml of sterile air into the back to generate the air pouch. After 3 days, another 3 ml of sterile air was injected into the pouch. After 3 days, 1 mg of CS in 500 μl of endotoxin-free PBS was injected into the air pouch. Control animals received only 500 μl of endotoxin-free PBS. After 6 h, animals were euthanized and the air pouch was lavaged with 3 ml of PBS. CS promotion of implantable lung tumours LKR13 cells used in this study were kindly provided by Dr Tyler Jacks [28] . To establish LKR13 tumours [51] , 2 × 10 6 live LKR13 cells in presence of 2 mg CS particles were resuspended in 100 μl PBS, mixed with 100 μl matrigel (Corning) and injected s.c. into the right flank of naive 6–8–week-old BLT1 + / + Rag2 −/− and BLT1 − / − Rag2 −/− mice. Mice injected s.c. with LKR13 cells alone served as controls. Tumour growth was monitored two to three times per week, and tumour size was measured in millimetres using a caliper. Average tumour size was calculated by measuring two perpendicular diameters. Animals bearing tumours were euthanized when tumours reached a size of 15 mm in one of the two perpendicular diameters or earlier if tumours ulcerated or the animal showed signs of discomfort. Lung histopathology BLT1 +/+ K-ras LA1 and BLT1 −/− K-ras LA1 mice (105 days old) were analysed for lung tumour burden. Lungs were inflated with 10% buffered formalin and were then removed, fixed in 10% buffered formalin for 24 h and stored in 70% ethanol. Lung lobes were separated and processed, embedded in paraffin and serially sectioned. Mid-sagittal 5-μm serial lung sections (200 μm apart) were stained with haematoxylin and eosin and digitally scanned on Aperio ScanScope. Lung sections were analysed by an experienced pulmonary pathologist. Lung lesions (hyperplasia—H, adenomatous hyperplasia—AH and adenoma—A) based on the histological features [52] were enumerated on the entire lung section using the digital image. Digital images of lung sections were also used to analyse lung inflammation. Lung inflammation is quantified as the percentage of inflamed lung area to total lung area in haematoxylin and eosin-stained lung sections. Lung tissue macrophages in the sections were identified by immunohistochemistry. Sections were stained with 1:50 diluted Rat anti-mouse F4/80 antibody (clone CL:A3-1, cat.# MCA497G, AbD Serotec) at the Pathology Core Research Laboratory at University of Louisville, following the standard protocol. Five independent fields per mouse lung section were randomly selected for macrophage counting and average macrophages per field were represented. CS particles in the lungs sections were viewed under polarized light and lungs were semi-quantitatively scored on a scale of 1–3 for the amount of deposited particles. Immune cell identification by flow cytometry Leukocytes were collected from airways, air pouch or peritoneal cavity by lavage; from unlavaged whole lungs, LKR13 s.c. tumours, spleen or cultures of bone-marrow-derived macrophages (BMDMs) and mast cells. A single-cell suspension was obtained from whole lungs or s.c. tumours by digesting the tissue in an enzyme mixture consisting of collagenase A (2 mg ml −1 ) and DNase I (100 μg ml −1 ) for 1 h at 37 °C with occasional vortexing. The digested tissue was filtered through a nylon mesh, and the resultant cells were washed twice in PBS. In total, 2 × 10 6 cells in single-cell suspensions were incubated with F C -receptor-blocking antibody followed by staining with various cell surface marker antibodies from BD Biosciences (San Diego, CA) or BioLegend (San Diego, CA), following standard protocols. Flow cytometry data were acquired on FACS Calibur or FACS Canto (BD Biosciences) and analysed using Flowjo software (Tree Star). In the lung tissue and airways (BALF), leukocytes were identified as CD45 + cells, alveolar or lung macrophages as CD45 + FSC hi CD11c hi F4/80 + cells, neutrophils as CD45 + CD11c − Ly6G hi Siglec-F − cells, B cells as CD45 + FSC lo B220 + cells, CD4 cells as CD45 + FSC lo CD4 + and CD8 cells as CD45 + FSC lo CD8 + . In the peritoneal cavity, macrophages were identified as CD45 + FSC hi F4/80 + cells and neutrophils as CD45 + SSC hi Ly6G hi cells. In spleen, B cells were CD45 + FSC lo B220 + and T cells were CD45 + FSC lo CD3 + . Macrophages from bone marrow cultures were CD11b + F4/80 + and mast cells from bone marrow cultures were CD117 + FcɛR1 + . In the s.c. tumours, leukocytes were identified as CD45 + cells, macrophages as CD45 + FSC hi F4/80 + CD11b hi Ly6G lo cells, mast cells as CD45 + CD117 + FcɛR1 + and neutrophils as CD45 + SSC hi Ly6G hi cells. In air-pouch lavage fluid, leukocytes were identified as CD45 + cells, macrophages as CD45 + FSC hi F4/80 + CD11b hi Ly6G lo cells and neutrophils as CD45 + SSC hi Ly6G hi cells. Cytospin preparations of the air-pouch lavage fluid cells were also done using Shandon Cytospin centrifuge (Shandon Lipshaw) followed by staining with Hema-3 reagents (Fisher Scientific) according to the manufacturer’s recommendations. Isolation of lung mast cells and alveolar macrophages Cells obtained from pooled lung digests of four naive WT mice were treated with RBC lysis buffer (BD Biosciences), resuspended in DMEM containing 10% fetal bovine serum (FBS) and incubated at 37 °C. The non-adherent cells were transferred after 8 h into fresh tubes without disturbing the adherent (macrophages and fibroblast) cells. The non-adherent cells were then incubated with F C -receptor-blocking antibody followed by staining for CD45, CD117 and FcɛR1 in 5% BSA. Mast cells identified as FSC hi CD45 + CD117 + FcɛR1 + cells were sorted using BD FACS Aria III cell sorter. Purity of the cells was 95.3%. Whole-lung lavage from 10 naive WT mice were pooled, resuspended in DMEM containing 10% FBS and incubated at 37 °C for 4 h. The non-adherent cells were discarded and alveolar macrophages were obtained by dislodging the adherent cells, followed by staining for CD45 and F4/80 after blocking F C -receptors. Purity of the cells was 99.5%. Isolation and culture of primary murine cells BMMCs were prepared from 6–8-week-old mice of indicated genotypes. Briefly, bone marrow cells were flushed out and cultured in DMEM containing 10% FBS, 100 units per ml penicillin, 100 μg ml −1 streptomycin, 2 mM L-glutamine, 50 μM β-mercaptoethanol supplemented with 12.5 ng ml −1 recombinant Mouse stem cell factor (R&D # 455 MC, 10 μg ml −1 stock) and 10 ng ml −1 recombinant Mouse IL-3 (R&D #403-ML, 10 μg ml −1 stock). The bone marrow cells were plated at ∼ 1 × 10 6 ml −1 density in T-75-cm 2 flask containing 15 ml of medium. The non-adherent cells were transferred after 48 h into fresh flasks without disturbing the adherent (fibroblast) cells. The flasks were changed weekly or as needed to separate the non-adherent mast cells from the contaminating adherent cells. The medium was changed once a week with medium containing SCF, IL-3. The homogenous population of mast cells was visible after 4 weeks of culture and propagated further for 4 weeks. The purity of BMMCs derived from WT or various knockout mice was confirmed to be ≥99% by surface staining for mast cell-specific markers CD117 and FcɛR1. BMDMs were prepared from 6–8-week-old mice of indicated genotypes. Briefly, bone marrow cells were flushed out and cultured in DMEM containing 10% FBS, 100 units per ml penicillin, 100 μg ml −1 streptomycin, 2 mM L-glutamine and 50 μM β-mercaptoethanol supplemented with 100 ng ml −1 recombinant Mouse macrophage colony-stimulating factor (BioLegend). The bone marrow cells were plated at 0.6 × 10 6 ml −1 density in 100-mm tissue culture dishes containing 10 ml of medium. After 3 days, the medium was replaced by 10 ml of fresh growth medium and a homogenous population of macrophages was visible. The cultures were maintained for another 3 days before stimulation. The cells were found to be more than 99% pure as confirmed by surface staining for F4/80 and CD11b. Eight-week-old mice were injected intraperitoneally with 2 ml of 3% aged thioglygollate medium. Peritoneum was lavaged after 10 h or 4 days to obtain elicited neutrophils and macrophages, respectively. The purity of thioglycollate elicited neutrophils and macrophages; resident peritoneal macrophages were ≥95%. For CS stimulation assays, mast cells from various sources were plated at 0.3 million per well of 12-well tissue culture dishes in 400 μl of medium without FBS. Primary macrophages from various sources, splenocytes and neutrophils were plated at 0.3 million per well of 12-well tissue culture dishes in 400 μl of 1% FBS-containing medium. All primary cells were stimulated with 100 μg cm −2 of CS for 6 h. Primary macrophages from all sources were primed with 10 ng ml −1 of lipopolysaccharide (InvivoGen) for 3 h prior to CS stimulation. LKR13 and RAW264.7 cells were cultured in DMEM containing 10% FBS. For CS stimulation assays, 0.3 million cells were plated per well of 12-well tissue culture dishes in 400 μl of 1% FBS-containing medium. The cells were stimulated for 6 h with 120 μg cm −2 of CS. Whenever indicated RAW264.7 cells were pre-treated with 10 μM Zileuton (5-LO inhibitor) for 1 h. Cell migration assay Chemotaxis of 300.19 cells and thioglycollate-elicited peritoneal neutrophils was evaluated using 5-μm pore size Transwell filters (Corning Costar, Cambridge, MA). Briefly, 1 million cells in 100 μl of medium were loaded onto the upper chamber. The lower chamber was loaded with 600 μl of either medium alone or 0.3 nM LTB 4 or unstimulated RAW264.7 cell supernatants or 120 μg cm −2 of CS-stimulated RAW264.7 cell supernatants. After 3 h of incubation at 37 °C in 5% CO 2 , the upper chamber was removed and cells that migrated to the lower chamber was counted. LTB 4 and IL-1β quantification S.c. tumours were homogenized in 500 μl 1 × PBS buffer containing 10 μM Indomethacin using the Omni GLH general homogenizer. The homogenates were centrifuged at 14,000 g for 10 min and LTB 4 levels in the supernatants were quantified. The LTB 4 levels were normalized to the amount of protein in the supernatants measured using the Themo Sceintific Pierce BCA protein assay kit following the manufacturer’s instructions. LTB 4 in the tumour homogenate supernatant was expressed as pg mg −1 of protein. LTB 4 in cell culture supernatants, BALF, air-pouch lavage and s.c. tumours was measured using the LTB 4 EIA Kit (Cayman Chemical) according to the manufacturer’s instructions. IL-1β in cell culture supernatants was measured using the Mouse IL-1β ELISA MAX Standard Kit (BioLegend) according to the manufacturer’s instructions. Quantitative RT–PCR Total RNA from LKR13 cells, BMDMs and mast cells, s.c. tumours as well as lungs was isolated using an RNeasy Mini Kit (Qiagen) in accordance with the manufacturer’s protocol. RNA samples were treated with DNase (Qiagen) before reverse transcription with TaqMan reverse transcription reagents (Applied Biosystems) using random hexamer primers. Quantitative PCR analyses were conducted as described previously [53] using ‘power SYBR-green master mix’ (Applied Biosystems). Expression of the target genes was normalized to GAPDH and the relative fold changes were calculated using the delta CT method. The fold changes were displayed relative to the PBS (vehicle)-treated BLT1 +/+ samples or LKR13-injected BLT1 + / + Rag2 −/− group. Data were representative of tissues isolated from at least five different mice for each cohort or triplicate cell cultures. The GAPDH , IL-1β , TNF-α , CXCL1 , CXCL2 , CXCL3 , CXCL5 , CCL2 , CCL3 , CCL4 , CCL5 , CXCR1 , CXCR2 and CCR5 primers obtained from RealTimePrimers.com were used in this study. Microarray and data analysis Total RNA was prepared from mouse lung tissues as described above. The microarray was performed using Affymetrix GeneChipMouse Gene 1.0 ST Array according to manufacturer’s protocol at the University of Louisville genomics facility. The GeneChip-brand array comprised of over 750,000 unique 25-mer oligonucleotide features constituting over 28,000 gene level probes with an average of 27 probes per gene. Briefly, Total RNA was amplified and labelled following the Affymetrix (Santa Clara, CA) standard protocol for whole-transcript expression analysis, followed by hybridization to Affymetrix Mouse Gene 1.0 ST arrays. The arrays were processed following the manufacturer recommended wash and stain protocol on an Affymetrix FS-450 fluidics station and scanned on an Affymetrix GeneChip 7G scanner using Command Console 3.1. The resulting .cel files were imported into Partek Genomics Suite 6.6 and transcripts were normalized on a gene level using RMA as normalization and the background correction method. Contrasts in a one-way analysis of variance were set up to compare the treatment groups of interest. The fold changes in gene expression along with Affymetrix IDs and P values were uploaded onto MetaCore pathway analysis software. The fold change in cytokines, chemokines and their receptors were displayed relative to the PBS (vehicle)-treated BLT1 +/+ sample and represented in graphs. Data were representative of pooled lung tissue RNA isolated from three different mice for each group. The data from the array analysis has been deposited in the NCBI public access database ( http://www.ncbi.nlm.nih.gov/geo/query/acc.cgi?acc=GSE66985 ). Multiplex analysis Whole-lung lavage fluids from PBS- or CS-treated BLT1 +/+ K-ras LA1 and BLT1 −/− K-ras LA1 or BLT1 +/+ and BLT1 −/− mice were analysed for levels of various inflammatory proteins namely TNF-α, CXCL1, CCL3, CCL4 and CCL5. The analysis was performed following standard protocols at the Proteomics core facility of Medical University of South Carolina. Data analysis All data are analysed with GraphPad Prism4 Software, San Diego, CA, and expressed as the means±s.e. from at least three independent samples. Statistical difference among groups was analysed using the Mann–Whitney U -test ( in vivo ) or unpaired Student’s t -test ( in vitro / ex vivo , RNA analysis). Two-tailed P values of <0.05 were considered as significant. Accession codes. The microarray data have been deposited in the Gene Expression Omnibus database udner accession code GSE66985 . How to cite this article: Satpathy, S.R. et al. Crystalline silica-induced leukotriene B4-dependent inflammation promotes lung tumour growth. Nat. Commun. 6:7064 doi: 10.1038/ncomms8064 (2015).